High-fidelity spin entanglement using optimal control Precise control of quantum systems is of fundamental importance in quantum information processing, quantum metrology and high-resolution spectroscopy. When scaling up quantum registers, several challenges arise: individual addressing of qubits while suppressing cross-talk, entangling distant nodes and decoupling unwanted interactions. Here we experimentally demonstrate optimal control of a prototype spin qubit system consisting of two proximal nitrogen-vacancy centres in diamond. Using engineered microwave pulses, we demonstrate single electron spin operations with a fidelity F ≈0.99. With additional dynamical decoupling techniques, we further realize high-quality, on-demand entangled states between two electron spins with F >0.82, mostly limited by the coherence time and imperfect initialization. Crosstalk in a crowded spectrum and unwanted dipolar couplings are simultaneously eliminated to a high extent. Finally, by high-fidelity entanglement swapping to nuclear spin quantum memory, we demonstrate nuclear spin entanglement over a length scale of 25 nm. This experiment underlines the importance of optimal control for scalable room temperature spin-based quantum information devices. High-fidelity quantum operations, including gates, on-demand entangled state generation and coherent control in general, represent a fundamental prerequisite for all quantum information technologies such as error correction, quantum metrology and of course quantum information processing, wherein the hardware and its control must satisfy the DiVincenzo criteria [1] . A very promising class of quantum information devices are spin qubits in solids, such as phosphorus in silicon (Si:P) [2] , rare earth ions in a solid state matrix [3] , quantum dots [4] and defects in diamond or silicon carbide [5] , [6] . Although there have been recent experimental advances in increasing the number of coherently interacting qubits [7] , [5] , gate quality has been limited. Optimal control, often seen as a central tool for turning principles of quantum theory into new technology [8] , seems to be the only practical way to ensure functionality even in the light of device imperfections, and to overcome several impactful features found when scaling up the register size, such as unwanted cross-talk between control fields designed for individual qubit control. It is gradually being exploited in many other experimental settings, including ion traps [9] , optical lattices [10] , solid-state devices [11] , [12] , [13] and NMR [14] . Nitrogen-vacancy (NV) centres in diamond are unique and interesting building blocks for implementing solid state quantum technologies [15] , [16] , [17] , [18] , [19] , [20] , [21] , [22] , [23] , [24] , [25] , [26] . More precisely, each such block comprises the NV centre’s electron spin and the nuclear spins of the nitrogen and proximal 13 C nuclei, forming a small quantum register [27] . Even without optimal control, several hallmark demonstrations of their properties have been possible, including coherent single qubit operation and readout [28] , [29] , controlled qubit gates [30] , [24] and entanglement generation [5] , [25] , [26] , [27] , [31] at ambient conditions. NV centres have been shown to exhibit coherence times on the order of milliseconds in isotopically purified diamond [32] or through dynamical decoupling [33] , [34] . This has to be compared with coherent control in the nanosecond regime [35] . Particularly, the nuclear spins have proven to be a valuable resource for high-fidelity readout [27] , [36] , [37] and non-volatile memory [38] . As such, NV centre registers can act as a prototype for any other spin qubit system. For spin quantum registers, scalability can be achieved through coherent interaction between neighbouring nodes in arrays of fundamental building blocks. The most straightforward approach is to place the blocks sufficiently close to each other [39] , [40] and use the dipolar interaction between electron spins as a quantum bus. The effective magnetic dipolar interaction range is limited by the coherence lifetime (here:~2 ms) to about ~50 nm for electron spins and ~5 nm for nuclear ones. The readout method depends strongly on the system. While for Si:P single-spin readout is performed with single-electron transistors [2] , in the case of NV centres in diamond optical super-resolution techniques facilitate individual optical spin readout with nanometer-scale resolution [41] . In contrast to optical techniques, microwaves cannot be focused down to these length scales. Individual spin addressability via magnetic resonance can be achieved by separating the spins’ resonance frequencies, for example, by applying local magnetic field gradients (≈2 μT nm −1 ) or by exploiting different crystal field directions. Coherent control of individual electron and nuclear spins is then conducted via resonant mw and rf fields. The nuclear spins can be additionally controlled via their hyperfine interaction with the neighbouring electron spin; effectively, the electron spin state sets the axis and speed of nuclear Larmor precession [42] . Note that the dipolar interactions between spins are always on, and the unavoidably crowded spectrum leads to non-negligible control cross-talk. Consequently, it becomes challenging to perform strictly local operations. While all these are minor issues for standard spectroscopy techniques, the fidelity of quantum operations can be drastically affected, especially for repeated gate application. In this work, we demonstrate a decisive step towards mastering the aforementioned challenges by developing optimal control methods for solid state spin registers to markedly increase their utility. We explore a prototype of such a quantum register, operating at ambient conditions, based on two neighbouring NV centres in diamond. These fundamental building blocks each comprise one electron spin qutrit and one nuclear spin qubit. We implement optimal control on this system of 36 levels to realize a fully functional four-qubit register. 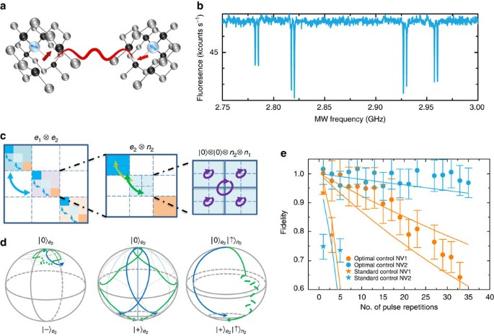Figure 1: Optimal control of a single qutrit. (a) Schematic of the NV-NV pair used in this work. (b) Optically detected magnetic resonance (ODMR) spectrum of the NV pair. The outer pairs of transitions correspond to NV1 and the inner pairs to NV2. The splitting within one pair of ≈3 MHz is due to the hyperfine coupling with the15N nucleus. Spin transitions of separate NV centres are separated by ≈30 MHz. (c) Concatenated representation of the 36 dimensions of the Hilbert spacecorresponding to two coupled NV centres. (left) Subsystemis shown with blue arrows illustrating electron spin manipulation on NV1 (bold, solid arrows) and its cross-talk on NV2 (dashed arrows). (centre) The subspaceis shown and green arrows of different tones illustrate the detuning due to hyperfine interaction. (right) The always-on nuclear spin precession by external static magnetic fields in subspaceis illustrated (curved arrows). The colouring of the squares denotes the different electron spin states,and. For NV2 this corresponds to blue, purple and light orange. For NV1 this corresponds to dark blue, light blue and orange. (d) Schematic Bloch sphere representation of the action of standard control (blue) and optimal control (green) considering the above mentioned effects. (left) Manipulation of spine1should not affect the state of spine2via cross-talk, (centre) despite hyperfine interaction the spine2should be inverted regardless of the state of nuclear spinn2, and (right) always on rotation of nuclear spinsn1,n2for electron spin statesshould be avoided if not exploited. (e) Repeated application of anotgate targeted on spine1, implemented using a standard π-pulse (stars) as compared with an optimized gate (filled circles). With an odd number of applications, the effect should always be the same (spin flipped fore1, unchanged fore2). The fidelity with respect to these target states is displayed for both spins (orange and blue). Where optimal control pulses allow for at least 20 repetitions without a significant loss of fidelity and negligible cross-talk within our measurement error, π-pulses show low fidelity and strong cross-talk already after the first gate application. Error bars are given by the photon shot noise of the measurement used to calculate the fidelity. High-fidelity single- and multiqubit operations are demonstrated ( Table 1 ). These include generating high-fidelity entanglement between the electron spins and entanglement storage in nuclear spin memory. The numerical control optimization simultaneously cancels cross-talk and unwanted dipolar couplings to a high extent. Our results will find further applications in any high-fidelity gate synthesis necessary for various scaling approaches devised so far (for example, refs 43 , 44 ). Table 1 Fidelity comparison. Full size table Optimal control Improving gate fidelity is a non-trivial task; the main reason for this being the high spectral density of individual qubit control fields. The interaction of a single microwave field with a spin can be described by the Rabi formula giving the probability p target for a spin flip into a target state. Here the Rabi frequency Ω is the strength of the applied mw field and Δ is the detuning of the mw frequency from the actual spin transition. While it seems that high-fidelity control of a single transition (that is, p target ≈1) can be achieved by a large ratio Ω/Δ, in the case of single-qubit gates on the electron spin (that is, irrespective of the nuclear spin state), the hyperfine interaction sets a lower bound for the detuning Δ and the spectral density sets an upper bound for Rabi frequency Ω to avoid cross-talk. In our particular case, the hyperfine interaction is ≈3 MHz and the spectral separation of individual NV transitions is ≈30 MHz (see Fig. 1b ). This limits the fidelity of a ‘standard’ single-pulse single-qubit not gate to F ≈0.9. During the finite duration of electron spin control, additionally, the nuclear spins undergo rotations dependent on the respective electron spin projection. While this will be exploited for nuclear spin control (see below), it further reduces the fidelity of single-pulse electron spin gates (see Fig. 1c ). These limitations can, however, be overcome using numerically optimized composite control sequences. Figure 1: Optimal control of a single qutrit. ( a ) Schematic of the NV-NV pair used in this work. ( b ) Optically detected magnetic resonance (ODMR) spectrum of the NV pair. The outer pairs of transitions correspond to NV1 and the inner pairs to NV2. The splitting within one pair of ≈3 MHz is due to the hyperfine coupling with the 15 N nucleus. Spin transitions of separate NV centres are separated by ≈30 MHz. ( c ) Concatenated representation of the 36 dimensions of the Hilbert space corresponding to two coupled NV centres. (left) Subsystem is shown with blue arrows illustrating electron spin manipulation on NV1 (bold, solid arrows) and its cross-talk on NV2 (dashed arrows). (centre) The subspace is shown and green arrows of different tones illustrate the detuning due to hyperfine interaction. (right) The always-on nuclear spin precession by external static magnetic fields in subspace is illustrated (curved arrows). The colouring of the squares denotes the different electron spin states , and . For NV2 this corresponds to blue, purple and light orange. For NV1 this corresponds to dark blue, light blue and orange. ( d ) Schematic Bloch sphere representation of the action of standard control (blue) and optimal control (green) considering the above mentioned effects. (left) Manipulation of spin e 1 should not affect the state of spin e 2 via cross-talk, (centre) despite hyperfine interaction the spin e 2 should be inverted regardless of the state of nuclear spin n 2 , and (right) always on rotation of nuclear spins n 1 , n 2 for electron spin states should be avoided if not exploited. ( e ) Repeated application of a not gate targeted on spin e 1 , implemented using a standard π-pulse (stars) as compared with an optimized gate (filled circles). With an odd number of applications, the effect should always be the same (spin flipped for e 1 , unchanged for e 2 ). The fidelity with respect to these target states is displayed for both spins (orange and blue). Where optimal control pulses allow for at least 20 repetitions without a significant loss of fidelity and negligible cross-talk within our measurement error, π-pulses show low fidelity and strong cross-talk already after the first gate application. Error bars are given by the photon shot noise of the measurement used to calculate the fidelity. Full size image For designing high-fidelity experiments, optimal control methods are gradually establishing themselves as valuable means to get the most out of an actual quantum experimental setting [45] , [46] . The general scenario involves minimizing a cost functional under the constraint that the system follows a given equation of motion. For state transfer or quantum gate synthesis in a closed system (neglecting decoherence for the moment), this amounts to the controlled Schrödinger equation. The control sequence is usually taken to be piecewise constant, so the pulse shapes can easily be fed to a digital pulse shaper. With these stipulations, effecting a desired quantum gate is (in principle) a standard task that can be conveniently addressed, for example, by the GRAPE [47] optimization algorithm in the DYNAMO numerical optimal control toolbox [48] . To handle non-idealities like cross-talk, we use a modified rotating wave approximation (RWA), taking sufficiently slowly rotating Hamiltonian components into account in addition to the static ones (see Methods). Our optimization framework also allows for Markovian [49] and non-Markovian [50] relaxation to be included. The final quality of the optimized control is of course limited by any deviation between the equation of motion used and the actual physics of the system. Please note that optimal control systematically goes beyond strict adiabaticity. This is of utmost importance in a dense spectrum of spin transitions of a potentially much larger register where it is almost impossible to avoid cross-talk effects. More precisely, for those unwanted transitions that are significantly detrimental to achieving the target, it suffices that they are effectively undone or refocused at the end of the control sequence, while intermediately they can be allowed for. While a paper-and-pen analysis of how this scales in dozens of qubits seems daunting, recursive use of optimal-control-based building blocks (of say up to 10 qubits) has proven promising [51] . The NV diamond spin system Our experimental system consists of two 15 NV centres separated by a distance of 25±2 nm, with an effective mutual dipolar coupling of v dip =4.93±0.05 kHz (ref. 5 ) (see Fig. 1a ). Each NV centre has an electron spin-1 (denoted S ) and a 15 N nuclear spin-1/2 (denoted I ), hence the system exhibits (3·2) 2 =36 energy levels in total. We label the m S =+1,0,−1 eigenstates of the S z spin operator with the symbols (+,0,−), and the m I =+1/2,−1/2 eigenstates of I z with (↑,↓). We use the states of the electron spin qutrit as an effective qubit and as an auxiliary state. Individual addressing of both NVs’ spin transitions is realized by different crystal field directions and proper magnetic field alignment resulting in a spectral separation of ≈30 MHz between the individual NV transitions (see Fig. 1b ). Although the crystal field and the external magnetic field are not parallel, spin states remain approximate eigenstates because of the much stronger crystal field along the NV axis. The hyperfine interaction of spin states with the 15 N nuclear spin aligns the latter along the NV axis and splits and by 3.01 MHz allowing for electron spin operations controlled by the nuclear spin (see Fig. 1b ). While the product states are approximate eigenstates and form the computational basis of each individual NV centre, the auxiliary states are not eigenstates and therefore facilitate electron spin-controlled nuclear spin rotations. Therefore, it is preferable to choose as qubit levels and use the as ancilla level for nuclear spin control. By this choice also unwanted electron-nuclear spin dynamics are suppressed [5] , [52] . Please note that the spin transition frequencies of the two individual NV centres are sufficiently far detuned (30 MHz) to avoid mutual flip-flop dynamics induced by the dipolar interaction (5 kHz). Instead, a decoupling sequence is used to realize a controlled phase gate among the two NV centres. The dephasing times of NV1 are μs and T 2dq =150±17 μs, and those of NV2 are μs and T 2dq =514±50 μs. The coherent manipulation of quantum states is separated from the optical readout process. There is no need for instantaneous readout after gate application. Hence coherent control of individual spins might be performed in a serial manner. Since individual optical addressing is challenging [41] at this short distance, here the readout is performed simultaneously on both NV centres. Therefore, the observed fluorescence is correlated with the sum of populations in the states of both NV centres. Individual spin state readout is achieved by local spin operations and repeated readout (see Supplementary Methods ). Optimal control with spin qubits Before implementing optimal control, a proper characterization of the spin Hamiltonian and the control fields is essential. This includes hyperfine interaction strengths, Zeeman shifts and control field transfer functions. In particular, the response of the NV electron spin to different frequencies and amplitudes of the control field is calibrated, compensating for non-linearities and spectral inhomogeneities. To compare standard and optimal control, we repeatedly apply a not gate to the electron spin of NV1 interrupted by a small free evolution time (see Fig. 1e ). First, the system is initialized into the state . If the applied gate is perfect, the state of NV1 always results in and that of NV2 in , neglecting decoherence. However, for standard control with rectangular time-domain pulses with Ω Rabi =10 MHz, the experimental results show a fast decay of population in for NV1 and a strong cross-talk effect on NV2 (that is, decrease of population in ) ( Fig. 1e ). In contrast, for optimal control the decay is much slower and almost no cross-talk is observed for 35 applications of the not gate. To quantify the precision of optimal control, we use a randomized benchmarking protocol and assume independent error sources for all applied optimal gates. A fidelity between 0.9851 and 0.9920 for the optimal not gate on NV1 and 0.9985 for the identity gate on NV2 are achieved by fitting the experimental results. Electron-nuclear spin operations The 15 N nuclear spins couple to magnetic fields much more weakly than the NV electron spins, and consequently have much longer coherence times. Therefore, they are ideal long-lived storage qubits [38] , which are easily integrated into a register via their hyperfine coupling to the electron spin. Various methods have been worked out for controlled nuclear spin operations. A particularly convenient one utilizes hyperfine interaction between electron and nuclear spins. To this end, the state acts as an ancilla level for nuclear spin manipulation. In contrast to , state exhibits no hyperfine coupling to the nuclear spin. Therefore, in state the nuclear spin is mainly susceptible to the external magnetic field and consequently undergoes Larmor precession around it with the angular frequency , where γ N is the nuclear gyromagnetic ratio. More precisely, the latter field is an effective one, where η describes the enhancement due to dressed nuclear-electron spin states [42] , [52] . In the current experiment, this effective field is almost perpendicular to the NV axis (see Methods). Therefore, the precession is a coherent oscillation between states and , which realizes a fast controlled rotation gate on the nuclear spin. Having at hand controlled rotations for electron and nuclear spins, we can design a partial swap gate ( pswap , exchanging the states and ) for quantum information storage. The standard approach is a sequence of rectangular time-domain pulses ( Fig. 2a ). However, the imperfections of each operation will accumulate and largely reduce the performance of the gate. We define the storage efficiency as the ratio of qubit coherences after and before storage and retrieval. For the standard pswap gate, we found the storage efficiency to be Eff std =0.50±0.07, which is mainly limited by cross-talk. With optimal control, we tailored a pswap gate with a significantly better performance compared with the standard approach ( Fig. 2c ). A storage efficiency of Eff opt =0.89±0.01 was measured. Eff opt is limited by decoherence during the pswap operation. The oscillation of the storage efficiency shown in Fig. 2c reveals the Ramsey oscillation of the nuclear spin due to the axial Zeeman shift with . 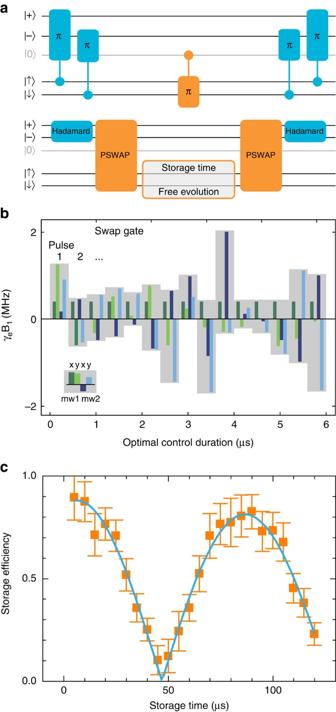Figure 2:Pswapgate between electron spin and nuclear spin. (a) Quantum wire diagrams for (top)pswapgate between the statesandvia standard control, utilizing the auxiliary state, and (bottom) creation, storage, retrieval and readout of a superposition state employing an optimizedpswapgate. (b) Optimal controlpswapgate consisting of 15 rectangular pulses (grey bars) each 0.4 μs long. Each pulse has two frequency components, corresponding to transitions(mw1, green) and(mw2, blue). In addition, each frequency component (mw1, mw2) has an in-phase and an out-of-phase amplitude (dark, bright). All four contributions to a single pulse are applied simultaneously during the whole pulse duration. (c) The retrieved superposition state reveals the free evolution during quantum state storage. Here we show thecomponent of the stored coherence. The Larmor precession of the nuclear spin superposition state leads to a phase accumulation. Error bars are given by errors of the fit of the phase amplitude and the shot noise of the reference measurement. The blue line is a fit of thecomponent taking an exponential decay due to the electron spin life time into account. Figure 2: Pswap gate between electron spin and nuclear spin. ( a ) Quantum wire diagrams for (top) pswap gate between the states and via standard control, utilizing the auxiliary state , and (bottom) creation, storage, retrieval and readout of a superposition state employing an optimized pswap gate. ( b ) Optimal control pswap gate consisting of 15 rectangular pulses (grey bars) each 0.4 μs long. Each pulse has two frequency components, corresponding to transitions (mw1, green) and (mw2, blue). In addition, each frequency component (mw1, mw2) has an in-phase and an out-of-phase amplitude (dark, bright). All four contributions to a single pulse are applied simultaneously during the whole pulse duration. ( c ) The retrieved superposition state reveals the free evolution during quantum state storage. Here we show the component of the stored coherence. The Larmor precession of the nuclear spin superposition state leads to a phase accumulation. Error bars are given by errors of the fit of the phase amplitude and the shot noise of the reference measurement. The blue line is a fit of the component taking an exponential decay due to the electron spin life time into account. Full size image Entanglement generation So far we have demonstrated coherent control within one NV centre node. However, scalability arises from coherent interaction of neighbouring NV nodes. The two NV centres of our register interact very weakly compared with their mutual detuning owing to Zeeman interaction. Thus, they only influence the phase accumulation on the other NV. To generate an entangled state, we therefore design and apply a controlled phase gate. Specifically, after initialization to , a local superposition state is created on both NV centres. Free evolution under the term of the Hamiltonian will then make the states accumulate a relative phase , where τ is the evolution time, effecting a non-local phase gate, which entangles the electron spins. μs will yield , at which point the state can be locally mapped into the Bell-type entangled state : To protect the phase accumulation from decoherence and possible couplings to other spins and thus achieve a higher fidelity, we additionally implement a Hahn echo π pulse in the middle of the free evolution period (see Fig. 3a ). Phase disturbances due to any quasi-static detuning (for example, hyperfine interactions with 15 N nuclei or slow magnetic field variations) are dynamically decoupled by the echo, allowing for a T 2 -limited gate fidelity. Taking into account the modest coherence time of NV1 ( T 2dq =150±17 μs) and the initial spin polarization (here 0.97 for each electron spin), the theoretical upper bound for the gate fidelity is F lim ≈0.849, which is in agreement with our measurement results. In the previous work on generating entanglement between two NV centres [5] , the fidelity was severely limited by pulse errors in the 16 local π and π/2 pulses used in the sequence, reducing it down to F std =0.67±0.04. By replacing these 16 rectangular mw pulses by just three numerically optimized local gates, we were able to improve the fidelity up to F opt =0.824±0.015, which reaches the limit set by decoherence and initialization fidelity (see Fig. 3b ). 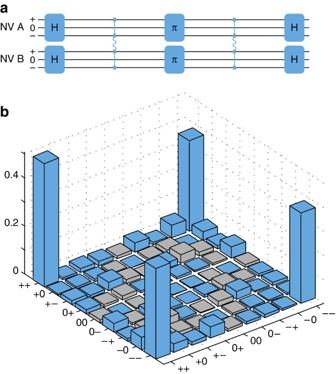Figure 3: Electron spin entanglement. (a) Quantum wire diagram of the entanglement sequence. (b) Density matrix of the created Bell state(F=0.824±0.015). The blue columns represent measured values. Please note that except for the main four columns representing the entangled state and the entriesand, all values are consistent with the shot noise of the measurement process. The grey columns are upper bounds given by the measured main diagonal entries and the requirements for a physical state. Figure 3: Electron spin entanglement. ( a ) Quantum wire diagram of the entanglement sequence. ( b ) Density matrix of the created Bell state (F=0.824±0.015). The blue columns represent measured values. Please note that except for the main four columns representing the entangled state and the entries and , all values are consistent with the shot noise of the measurement process. The grey columns are upper bounds given by the measured main diagonal entries and the requirements for a physical state. Full size image Entanglement storage Finally, we shall demonstrate entanglement storage on the nuclear spins using the pswap gate introduced above. To this end, a control sequence was optimized to execute simultaneous pswap gates on both NV centres yielding a storage efficiency of Eff opt =0.92±0.07 (compared with Eff std =0.39 achieved with standard pulses in previous work [5] ). The fidelity of the entangled state after storage and retrieval is F opt retrieved =0.74±0.04. It is important to note that during the spin state storage the two remote nuclear spins are entangled. Using reconstructed electron spin density matrices before, during and after the entanglement storage (presented in Fig. 3b and Supplementary Fig. 1 ), we can estimate the fidelity of the nuclear spin state to be F opt nuclear =0.819. The corresponding estimated density matrix of the entangled nuclear spins is shown in Fig. 4 . The state clearly fails the Peres-Horodecki criterion [53] (having a negativity of N nuclear ≈0.32), demonstrating its entanglement. Please note that during entanglement storage the nuclear spins are in a fairly pure entangled state, while the electron spins are in a mixed unentangled state due to the pswap gate between initialized electron spins and nuclear spins in a thermal state. Therefore, no postselection is necessary. To quantify the entanglement E ( ρ ) in our states, we numerically minimized the relative entropy by sampling over separable states σ (ref. 54 ), yielding E electron ≈0.37 and E nuclear ≈0.23 (out of the ideal ). This demonstrates a significant improvement of the NV-NV electron spin quantum entanglement in comparison with standard control, yielding only E std ≈0.16. 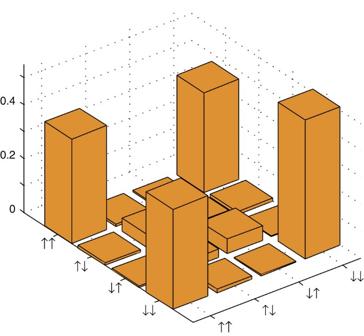Figure 4: Nuclear spin entanglement. Using optimal control, we have swapped the entangled electron spin state onto the nuclear spins (F=0.819). The orange density matrix represents the entangled Bell stateof the two remote nuclear spins. Please note that since the entanglement was created on the electron spins and transferred to nuclear spins usingpswapgates, no polarization or postselection is necessary to achieve nuclear spin entanglement. Figure 4: Nuclear spin entanglement. Using optimal control, we have swapped the entangled electron spin state onto the nuclear spins (F=0.819). The orange density matrix represents the entangled Bell state of the two remote nuclear spins. Please note that since the entanglement was created on the electron spins and transferred to nuclear spins using pswap gates, no polarization or postselection is necessary to achieve nuclear spin entanglement. Full size image In conclusion, we have demonstrated that the implementation of optimal control is a prerequisite for the realization of spin-based quantum information technology. The implementation itself is perhaps more challenging than in many other types of quantum systems due to the high level of cross-talk present in a multi-spin system. Such cross-talk has been identified as a limiting feature that needs to be overcome to make spin-based registers scalable. The present study offers strong supporting evidence that this challenge can indeed be overcome by optimal control. Especially for the nuclear spin storage (and thereby nuclear spin entanglement), cross-talk becomes a major issue. Here, an entanglement pswap fidelity larger than 0.94±0.03 is demonstrated, enabling meaningful entanglement storage and nuclear spin entanglement protocols. In this setting, our work may thus be envisaged as a breakthrough, where it was demonstrated that optimal control is an indispensable tool to achieve the combination of several highly demanding tasks simultaneously: high-end control of transitions in a crowed spectrum with 36 energy levels; suppression of cross-talk; creation of entanglement between distant nuclear spins with different quantization axes via control of electron-nuclear interactions on several timescales; and decoupling from unwanted interactions. Our control methods, though tailored for NV centres, can easily be transferred to other types of experimental systems as well. Thus, they are anticipated to find wide application. At the moment, the performance is mainly limited by the coherence times of the electron spins. However, this is a material property and long coherence times for artificially created NV centres have been demonstrated in isotopically purified diamond [55] . Recent advances in implantation techniques (that is, low energy mask implantations [39] ) as well as coherence time extension by growing an additional layer of diamond over the implanted NVs [40] will pave the way for a high-yield chip size fabrication of NV arrays. The methods developed in this work will play a crucial role in making the control of such spin arrays feasible. The control fidelity could be further improved by robust control sequences, which can automatically compensate for small magnetic field, temperature and control power fluctuations. Since the achieved control fidelity depends on the accuracy of the simulation used in optimization, accurate measurement of the system parameters (for example, the hyperfine tensor) is of paramount importance. In principle, the pulses could also be improved using closed-loop optimization where measurement data are immediately fed back to the optimizer to improve the pulses without full knowledge of the system [46] , [56] . Sample characteristics The diamond sample is grown by microwave-assisted chemical vapour deposition (CVD). The intrinsic nitrogen content of the grown crystal is below 1p.p.b. and the 12 C content is enriched to 99.9%. 15 N ions were implanted with an energy of 1MeV through nano-channels in a mica sheet. A characterization of this method was published recently [7] , [5] . Measurement setup The two NV centres of this work are optically addressed by a home-built confocal microscope. Microwave radiation was guided to the NV centres of interest using a lithographically fabricated coplanar waveguide structure on the diamond surface. Microwave control was established with an home-built IQ mixer and an arbitrary waveform generator (Tektronix AWG 5014C) to generate arbitrary microwave amplitudes, frequencies and phases. With the microscope and mw devices optically detected magnetic resonance (ODMR) of single NV electron spins is performed. To this end, a laser is used to initialize the electron spin into its state by laser excitation and subsequent decay. Next, the spin is manipulated by mw fields. Finally, the fluorescence response to a next laser pulse reports on the spin state (that is, low level for and high level for ). Magnetic field alignment The S =1 electron spin of the NV centre experiences a strong crystal field of about 100 mT along the centre's symmetry axis, splitting apart the levels from . As the symmetry axis has four possible orientations in a diamond crystal lattice, NV centres might differ in crystal field direction as for the present NV pair. A small magnetic field is used to lift the remaining degeneracy of to guarantee individual addressing of spin transitions. Here, using magnetic field coils, a magnetic field of 3.41 mT with an angle of about 24° to the NV1 axis and 125° to the NV2 axis was applied. To have no effect from the different charge states of the NV centre charge state pre-selection was implemented [57] . Simulating the NV system A single 15 NV − centre in a static magnetic field B 0 = B 0 u 0 has the Hamiltonian where S and I are the dimensionless spin operators for the electron pair and the 15 N nucleus, respectively, quantized along the NV symmetry axis. Lattice strain has been neglected. Δ≈2.87 GHz is the zero-field splitting. The anisotropic (but axially symmetric) hyperfine coupling coefficients are A xx = A yy ≈3.65 MHz and A zz ≈3.03 MHz (ref. 58 ). The Larmor frequencies are defined as ω I :=− γ I B 0 , where γ I is the gyromagnetic ratio of the spin (electron or nuclear). In a typical experiment ω e ≈100 MHz. The system can be controlled using oscillating magnetic fields of the form where are the carrier frequencies (in the microwave region). The amplitudes B k and the phases can be changed in time to steer the system. The unit vectors u k , representing the polarization of the control signal, are determined by the antenna setup. In our case u k || [001]. The control fields add additional Zeeman terms for both the electron and the nuclear spins: where Ω k ( t ) is the driving Rabi frequency, C k is the corresponding control operator and is the length of the perpendicular component of u k . The reason for this normalization is that when B 0 is aligned with the NV axis, only the perpendicular component of the control field drives a population transfer. The system of two coupled NV centres is then described by the Hamiltonian where H NV1 and H NV2 are the Hamiltonians of the individual NV centres, NV 1 and NV 2, respectively, and H int describes the dipolar interaction between them: The two NV centres are separated by a distance of r =25±2 nm, and the strength of the dipole–dipole interaction between them is found to be v dip =4.93±0.05 kHz. Because of the strong, local zero field splitting and Larmor terms, the effect of all the H int terms but the S z 1 S z 2 one are strongly suppressed and may be neglected. Thus, we obtain The dipolar interactions between S 1/2 and I 2/1 , and between the two nuclear spins are weaker by factors of and , respectively, and can be safely ignored. In the experiment, the two NV centres have different axis orientations, [111] and , which makes them individually addressable even in a uniform magnetic field. The static magnetic field B 0 makes the angle θ 1 ≈0.133 π with and the angle θ 2 ≈0.695 π with . Such alignment leads to considerable hyperfine splitting in the m S =0 level (see Fig. 5 ) due to a small admixture of levels m S =±1, which leads to small magnetic moment roughly perpendicular to the NV axis. As the hyperfine field at the nitrogen nucleus for the m S =0 level is almost perpendicular to the ones for levels m S =±1 different nuclear spin quantization axes arise. The latter can be utilized for coherent nuclear spin control in the in m S =0 subspace via the electron spin, for example, to perform a (partial) swap operation between the electron spin and the nuclear spin. 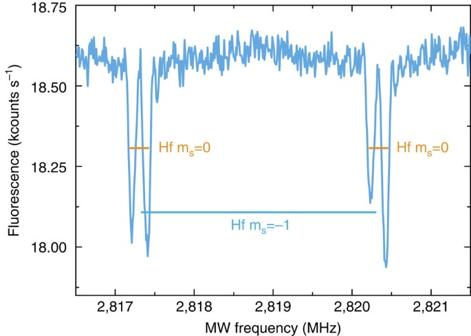Figure 5: High-resolution ODMR spectrum. The spectrum was recorded for thems=0→ms=−1 transition of NV2. Figure 5: High-resolution ODMR spectrum. The spectrum was recorded for the m s =0→ m s =−1 transition of NV2. Full size image Calibration Once the Hamiltonian parameters are known (by fitting them to the measured hyperfine ODMR peaks such as the ones in Fig. 5 ), we determine the (in general nonlinear) dependence between the amplifier setting α and the corresponding driving Rabi frequency Ω k for each carrier frequency separately. This is done by finding, for a set of values of α, the Ω k :s that yield the best match between simulated and measured single driving data, and doing, for example, monotonous cubic spline interpolation between the points. Rotating wave approximation We use two independent methods to simulate our system. Both yield high-fidelity pulses. One approach is to apply perturbation theory first to remove non-secular terms in the free evolution Hamiltonian [52] . When moving into a rotating frame the control Hamiltonian still has time-dependent terms, which can be made time-independent by using Floquet theory [59] . The second approach directly employs the rotating wave approximation and drops any terms with a small amplitude-to-rotation-frequency ratio. Here, we will describe the second method in detail. A rotating frame is an interaction picture defined by a time-independent, typically local, Hamiltonian H 0 . Given a system with the Hamiltonian H , we have in the Schrödinger picture . We then define the interaction picture ket At t =0, the rotating frame coincides with the lab frame. The corresponding transformation for operators is . Assume H 0 has the spectral decomposition , where ω k are unique and arranged in increasing order, and the orthogonal eigenspace projectors P k sum to identity. Now Assume that the system Hamiltonian is of the form where the carrier frequencies by convention. The rotating frame Hamiltonian is given by where δ ab := ω a − ω b , and we have further defined and . We use equation (12) to approximate the rotating frame Hamiltonian H ′ using the static term and a small number of slowly rotating terms. For each carrier frequency, all the terms that rotate at the same frequency ω (collected in the ordered pair index set Q ( ω )) are added together and retained if where s =300 is a cutoff parameter. The maximum control amplitude Ω max is chosen such that no fast mode is kept. We apply the control microwaves at four distinct carrier frequencies, each in the centre of the observed hyperfine peaks of a single-NV or transition. A convenient rotating frame is thus obtained by choosing H 0 to consist of the electron Zeeman and zero-field splitting terms, which makes the highest-magnitude control terms static. However, because of the relatively high spectral transition density in the NV-NV system, we will have some cross-talk, manifesting itself as non-negligible slowly rotating terms in the rotating frame Hamiltonian H′ ( t ), which need to be taken into account. Since an off-axial B 0 field makes H 0 slightly non-diagonal, the U 0 ( t ) transformation does not keep our observable perfectly invariant in time. This introduces a small additional error to the measurement. Numerical pulse optimization To implement a high-fidelity quantum gate G , that is, a specific unitary propagator of the system, we resort to optimal control techniques. The procedure involves defining an equation of motion for the system (in our case the Schrödinger equation in a rotating frame under the Hamiltonian in equation (6)), a set of control fields (the driving Rabi frequencies Ω k ( t ) and the phases in equation (5)), and a cost functional to be numerically minimized. For reasons of computational efficiency and ease of implementation, the control fields are taken to be piecewise constant in time. The cost functional is simply the error function where U ( T ) is the propagator obtained by integrating the Schrödinger equation of the system from 0 to T under the control sequence, and D the total dimension of the system. This choice of error function automatically absorbs unphysical global phases. In some cases, we are only interested in what happens to a specific subsystem, that is, we wish to obtain a propagator of the form where G is the gate to be implemented and W is an arbitrary unitary. The fact that we do not care what happens to the other subsystem(s) as long as the total propagator remains factorizable can make the optimization task much simpler. In this case the appropriate error function is where the trace norm is given by the sum of the singular values of A . It is easy to see how this reduces to equation (14) when the second subsystem is trivial. Because of the rapid oscillation of the control Hamiltonian equation (5), it is much faster to perform the integration in a suitable rotating frame, discarding all the non-static terms in the rotating frame Hamiltonian and thus making it time independent. This way we may utilize the GRAPE [47] algorithm to efficiently compute the gradient of the error function and a standard optimization algorithm (such as BFGS) to minimize it, using a customized version of the DYNAMO [48] optimization framework. However, this is an approximation that does not take into account cross-talk, which in our case can be significant. To push the gate fidelity higher, it needs to be accounted for. Hence, we only use the fast, rough method in the initial phase of the optimization. Once the gate error is low enough, we switch over to a more accurate time-dependent rotating frame Hamiltonian, which includes slowly rotating terms representing the most significant cross-talk components. The fidelities of the control sequences obtained in this way are ultimately limited by the accuracy of the simulation, the approximations used, and decoherence. The specific decoherence mechanisms can also be included in the optimization, but in our scenario (generation of full quantum gates) we did not deem it worthwhile. How to cite this article: Dolde, F. et al. High-fidelity spin entanglement using optimal control. Nat. Commun. 5:3371 doi: 10.1038/ncomms4371 (2014).